Edge dislocation slows down oxide ion diffusion in doped CeO2by segregation of charged defects Strained oxide thin films are of interest for accelerating oxide ion conduction in electrochemical devices. Although the effect of elastic strain has been uncovered theoretically, the effect of dislocations on the diffusion kinetics in such strained oxides is yet unclear. Here we investigate a 1/2<110>{100} edge dislocation by performing atomistic simulations in 4–12% doped CeO 2 as a model fast ion conductor. At equilibrium, depending on the size of the dopant, trivalent cations and oxygen vacancies are found to simultaneously enrich or deplete either in the compressive or in the tensile strain fields around the dislocation. The associative interactions among the point defects in the enrichment zone and the lack of oxygen vacancies in the depletion zone slow down oxide ion transport. This finding is contrary to the fast diffusion of atoms along the dislocations in metals and should be considered when assessing the effects of strain on oxide ion conductivity. Strain engineering offers a new route to tune the reaction and transport kinetics in oxide materials [1] by altering the inherent energy landscape of reactions, as demonstrated also for metals [2] , [3] and for polymers [4] , [5] . Strain can be induced in a material by lattice mismatch at the interface of a thin film with a substrate or with neighbouring layers (such as in multilayer composites). The lattice mismatch can be accommodated as elastic strain or as a combination of elastic and plastic strain. A high density of dislocations (two orders higher than those in bulk) can be found at the interface of thin films [6] , [7] , [8] upon relaxation of elastic strain. This high density of dislocations makes the study of their effect on the properties of the material of paramount importance. The elastic strain effects in oxides have been extensively studied for transport [9] , [10] , [11] , (electro)catalytic activity [12] , [13] , [14] and multiferroic properties [15] , [16] . On the other hand, only a few recent studies directly assessed the potential role of dislocations on the electrical [17] , [18] , magnetic [19] and chemical [20] , [21] properties of oxides, probably because of the intrinsic difficulty in studying these extended defects one at a time with high spatial resolution. Elastic strain is considered as a new knob to enhance the performance of oxide electrochemical devices, including solid oxide fuel cells (SOFCs) [9] , [10] , [11] , photocatalysts [22] , batteries [23] , electrolysers [24] and redox-based resistive memories [25] , by accelerating ion conduction. However, in most of these studies, the influence of strain was interpreted in terms of elastic strain alone, while plastic strain, that is, strain accommodated by dislocations, has been overlooked. In metals, dislocations are known to be fast diffusion paths due to their open space and low coordination environment [26] , [27] . This phenomenon has been called fast pipe diffusion (orders of magnitude faster than that in bulk). Because of what is known in metals, dislocations have been therefore suggested to enhance ionic conductivity in oxides as well [28] , [29] , [30] . For example, Sillassen et al. [28] have observed 3.5 orders of magnitude acceleration in the ionic conductivity for a 8.7 mol.% yttria-stabilized zirconia (YSZ) epitaxial film on MgO substrate. They attributed this enhancement qualitatively to a combination of misfit dislocations and elastic strain at the interface. Contrary to that example, Li et al. [31] have studied a YSZ/Gd 2 Zr 2 O 7 (YSZ/GZO) multilayer structure, which was said to be dislocation free. They found that YSZ presents a higher conductivity on GZO compared with thin YSZ films on CeO 2 , where dislocations are present. Li et al. [31] suggested that the relaxation of elastic strain brought by dislocations does not enhance ionic conductivity. Atomistic simulations [32] of a hetero-interface with a density of dislocations between CeO 2 and YSZ also showed that the oxygen diffusion coefficient is not enhanced within the interfacial region. However, because of the irregular network of dislocations in that model, the influence of individual dislocations was not accessible one at a time to see the diffusion along and across the dislocation lines. In such complex simulations, it is also not clear whether dislocations or other factors, such as interface chemistry, affect ionic conductivity primarily. Because of the limited number of studies (with contradictory results), it appears unclear whether the concept of pipe diffusion can be applied to oxide ion conductors at all. Indeed, previous experimental studies [33] and numerical calculations [34] of grain boundaries in ceria (which also present an open structure and low coordination environment) shows that ionic conductivity at the grain boundary is lower than that in the bulk of this material. In summary, despite the importance of dislocations in oxide thin films and chemo-mechanics of materials, the fundamental mechanisms by which a dislocation has an impact on the ionic diffusivity in these doped and/or reducible oxides are unknown. The aim of this study is to provide an atomistic view of how dislocations alter the formation, distribution and mobility of oxide ion defects. For this purpose, an ½<110>{100} edge dislocation is studied as a model system in reduced or doped ceria. Ceria is a known fast oxide ion conductor, with an oxygen-vacancy-mediated transport mechanism [35] . The highest ionic conductivities are observed when it is doped with trivalent cations, such as Gd, Sm and Y [36] . For this reason, it has been used as an electrolyte in SOFCs and, recently, its use as an anode or cathode material has also been suggested [36] , [37] . Finally, ceria is also widely used in catalysis [38] and is a state-of-the-art material for thermochemical water splitting [22] . The hypothesis of this study is that the interaction between dislocations and charged point defects, specifically dopant cations, reduced cerium cation (Ce 3+ ) and oxygen vacancies, can have an impact on the distribution and mobility of oxygen vacancies. Here, dislocations in reduced ceria (CDC), Gd-doped ceria (GDC), Y-doped ceria (YDC), Sc-doped ceria (SDC) and a hypothetical ceria model (which will be defined in Results) were investigated. For simplicity in the wording and analysis of the results, we will refer to Ce 3+ also as a dopant cation in the reduced ceria model here. We use a hybrid Monte Carlo and molecular dynamics approach (MCMD) [39] , [40] to predict and explain the impact of a dislocation on the distribution of charged defects and on the diffusion of oxygen. A subset of the results is also validated by density functional theory calculations corrected by the Hubbard model (DFT+U). A redistribution of dopant cations by accumulation or depletion of dopant cations in the strain field of the dislocation is found to take place due to the elastic energy minimization of the system. The cation redistribution is accompanied by the enrichment (depletion) of oxygen vacancies where the dopants or reduced cations enrich (deplete), mainly due to electrostatic interactions. Both the associative defect–defect interactions in the defect enrichment zone and the lack of charge carriers in the defect depletion zone slow down the oxide ion transport at the dislocation. These results show that edge dislocations are detrimental to the oxide ion conductivity of these materials. The mechanisms and outcomes demonstrated here are valid also for other doped and reducible oxides with a high concentration of defects. Simulated model system First, the simulated model system is displayed in Fig. 1 . 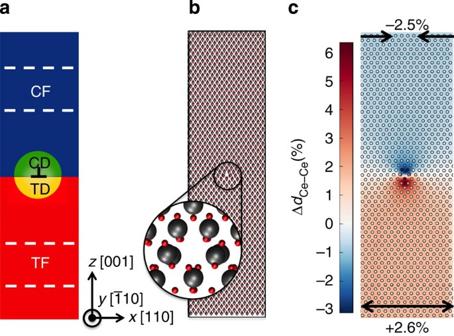Figure 1: Model of an edge dislocation in ceria. (a) The schematic of the super cell used in the atomistic calculations: a slab of ceria with an 1/2<110>{100} edge dislocation lying along theyaxis at the centre of the slab, with non-periodic boundaries along thez([001]) direction; the slab has a size of 6 × 2.7 × 22 nm3and 26,040 atoms in total. (b) The dislocation core structure. The grey spheres represent the cerium ions, while the red spheres represent the oxygen ions near the dislocation core. (c) The strain map, colour coded by the relative change of the local cation bond distance, ΔdCe–Ce=(ddisl−dbulk)/dbulk, whereddislanddbulkare the Ce–Ce bond distances in the model, with a dislocation and in the unstrained dislocation-free bulk model, respectively. Blue (negative) represents compressive strain and red (positive) represents tensile strain alongx([110]) direction far from the dislocation. The circles represent the cerium ions projected to thex–zplane. Figure 1a shows a schematic of a slab of ceria, with two {100} oxygen-terminated surfaces perpendicular to the z axis. The simulation box is periodic along the x and y axes, but non-periodic along the z axis. An 1/2 <110>{100} edge dislocation is introduced at the centre of the cell by removing a half-plane of atoms aligned at the [110] direction. The dislocation core structure ( Fig. 1b ) we obtained is in good agreement with the previous geometric description of the dislocation core [41] and computational models for other fluorite-structured oxide materials [42] , [43] . This edge dislocation has a non-uniform strain–stress field as mapped in Fig. 1c . The atomic level strains, denoted as Δ d Ce–Ce , are calculated by the relative change of the cation–cation bond distances in this model, Δ d Ce–Ce =(d disl − d bulk )/d bulk , where d disl and d bulk are the Ce–Ce bond distances in the model with a dislocation and in the unstrained dislocation-free bulk model. According to the strain field, the slab is divided into four regions, as shown in Fig. 1a : the tensile zones around and far from the dislocation (TD and TF, respectively) and the compressive zones around and far from the dislocation (CD and CF, respectively). The TD and CD regions have strongly distorted strain fields in the vicinity of the dislocation core. The TF and CF regions have uniaxial strain along [110] direction far from the dislocation because of the way we constructed this slab model by removing a half plane, while the model is periodic along the x and y directions. (More details for setting up the dislocation model are given in the Methods section.) Figure 1: Model of an edge dislocation in ceria. ( a ) The schematic of the super cell used in the atomistic calculations: a slab of ceria with an 1/2<110>{100} edge dislocation lying along the y axis at the centre of the slab, with non-periodic boundaries along the z ([001]) direction; the slab has a size of 6 × 2.7 × 22 nm 3 and 26,040 atoms in total. ( b ) The dislocation core structure. The grey spheres represent the cerium ions, while the red spheres represent the oxygen ions near the dislocation core. ( c ) The strain map, colour coded by the relative change of the local cation bond distance, Δ d Ce–Ce =( d disl − d bulk )/ d bulk , where d disl and d bulk are the Ce–Ce bond distances in the model, with a dislocation and in the unstrained dislocation-free bulk model, respectively. Blue (negative) represents compressive strain and red (positive) represents tensile strain along x ([110]) direction far from the dislocation. The circles represent the cerium ions projected to the x – z plane. Full size image We report the equilibrated distribution of Ce 3+ , Gd 3+ , Y 3+ , Sc 3+ and oxygen vacancies around the dislocation for the CDC, GDC, YDC and SDC models, respectively, in Fig. 2 . Here, all four models have the same bulk nominal dopant concentration of 8% and oxygen vacancy concentration of 2%. These distributions were equilibrated by means of MCMD calculations at 1,300 °C, while the total number of trivalent cations and vacancies were fixed in all simulations. The results indicate that both the dopants and the oxygen vacancies segregate significantly near the dislocation core, forming enrichment and depletion regions of 1–2 nm radius around the dislocation. For regions more than 3 nm away from the dislocation, the defects distribute uniformly and randomly as in the bulk without a dislocation. The compositional profile that arises around the dislocation depends on the elastic and electrostatic interactions among all types of defects, including the dislocation, dopant cations and oxygen vacancies, as will be de-convoluted below. The results reported below are also applicable for the models with 4% and 12% nominal dopant concentrations, which are documented in the Supplementary Fig. 1 . 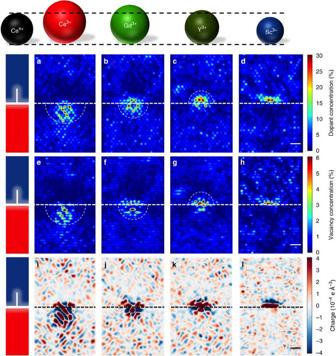Figure 2: Distribution of defects and net charge around the dislocation. Equilibrated distribution of (a–d) trivalent cations, (e–h) oxygen vacancies and (i–l) net charge in the (a,e,i) 8% CDC, (b,f,j) 8% GDC, (c,g,k) 8% YDC and (d,h,l) 8% SDC at 1,300 °C, with the dislocation located at the centre as shown in the schematic on the left for each row of results. The white dashed line marks the glide plane of the dislocation. The spheres represent qualitatively the relative size of dopant cations, Ce3+, Gd3+, Y3+and Sc3+, to the host cation, Ce4+. Scale bar, 1 nm. Figure 2: Distribution of defects and net charge around the dislocation. Equilibrated distribution of ( a – d ) trivalent cations, ( e – h ) oxygen vacancies and ( i – l ) net charge in the ( a , e , i ) 8% CDC, ( b , f , j ) 8% GDC, ( c , g , k ) 8% YDC and ( d , h , l ) 8% SDC at 1,300 °C, with the dislocation located at the centre as shown in the schematic on the left for each row of results. The white dashed line marks the glide plane of the dislocation. The spheres represent qualitatively the relative size of dopant cations, Ce 3+ , Gd 3+ , Y 3+ and Sc 3+ , to the host cation, Ce 4+ . Scale bar, 1 nm. Full size image Dopant segregation around the dislocation Dopants segregate to the dislocation core, as shown in Fig. 2a–d . An enrichment region appears near the dislocation, with a high dopant concentration of 25%–30% compared with the 8% of average concentration in all four models. This is accompanied by a depletion region on the opposite side of the dislocation, with a dopant concentration lower than 2%. The minimization of the elastic energy determines the location and geometry of the enrichment and depletion regions for the trivalent cations. For reduced ceria ( Fig. 2a ) and Gd-doped ceria ( Fig. 2b )), where Ce 3+ and Gd 3+ are larger than the host Ce 4+ , the dopants enrich at the tensile strain field of the dislocation, because placing the larger dopants in these expanded regions reduces the system energy. In contrast, Sc 3+ is smaller than Ce 4+ , and Sc 3+ cations enrich at the compressive region and deplete at the tensile region in the Sc-doped ceria ( Fig. 2d ). In the case of Y-doped ceria ( Fig. 2c ), the size of dopant cation Y 3+ is close to the host cation Ce 4+ and consequently, no significant enrichment or depletion is found in the strain fields of the dislocations. Instead, the Y 3+ accumulates at the two cation columns that directly face the dislocation core, but in the compressive part of the core. A bigger difference between the sizes of dopant cation and the host cation results in a stronger enrichment and depletion around the dislocation. As seen in Fig. 2a,b , the spatial extent of the segregation region in CDC is around 2 nm, larger than that in GDC, which is 1.5 nm. We note that the segregation regions follow the strain field shape of the edge dislocation and have a semi-cylindrical boundary for both the enrichment and depletion zones. The only exception is SDC, which has an enrichment region with an irregular shape. This is probably due to the significantly smaller radius of Sc, which leads to Sc clustering that overrides the effect of the elastic strain field. Extensive clustering of Sc cations in bulk ceria is known [44] . The geometry and location of enrichment and depletion zones may change for other types of dislocations in ceria, depending on their strain–stress field. Although an experimental validation of this prediction is not present in literature on the level of a single dislocation in ceria, we find evidence to cation segregation near extended defects in ceria, such as grain boundaries [33] , [45] , [46] and surfaces [47] , [48] . The thickness of the experimentally found segregation zone varies as 1–5 m, which is comparable to the segregation profile observed here. Furthermore, high-resolution transmission electron microscopy examination in other materials, in particular the interface of (Nd 0.35 Sr 0.65 )MnO 3 /SrTiO 3 , demonstrated that edge-type misfit dislocations allow for interdiffusion of cations within a semi-cylindrical boundary around the dislocation [7] , as also predicted for the dislocations of ceria in this work. The edge dislocation modelled in this paper can be different from misfit dislocations at the thin-film/substrate interfaces due to the local structure and chemical composition [49] . However, the key driver of cation and vacancy segregation around the edge dislocations in bulk ceria studied here is the strain field, which is also present around misfit dislocations. Therefore, it is reasonable to observe that the interdiffusion of cations around misfit dislocations at the (Nd 0.35 Sr 0.65 )MnO 3 /SrTiO 3 interface is similar to our prediction for dislocations in ceria. Such strong segregation of cations then impacts the oxide ion conductivity, as shown and discussed later. The qualitative description of the segregation profiles predicted and shown above for the 8% doped CDC, GDC, YDC and SDC are also valid for the models with 4% and 12% dopant concentrations, surveyed for CDC and GDC ( Supplementary Fig. 1 ). The size of the enrichment area does not exceed 2 nm in all cases, while local concentration of dopants is never higher than 30%. This implies that dislocations are not an infinite sink for dopant cations, but get eventually saturated, and always retain the fluorite structure. Oxygen vacancy segregation around the dislocation The segregation profile of oxygen vacancies matches that of the dopants around the dislocation, that is, oxygen vacancies enrich where the dopants enrich and they deplete where the dopants deplete. This can be seen by comparing Fig. 2a–d with Fig. 2e–h . In CDC and GDC the enrichment and depletion of oxygen vacancies and dopants are in the tensile and compressive fields, respectively, whereas in SDC the enrichment and depletion of these defects are in the compressive and tensile fields, respectively. In YDC, the enrichment of oxygen vacancies is localized right on the dislocation core, nearest to the columns where Y 3+ cations have accumulated. In the previous section, we have concluded that the segregation of the dopants to the dislocation strain fields is driven primarily by elastic energy minimization, similar to that in metals. Solely based on elastic energy arguments, one would expect the vacancies to be all in the compressive strain fields of the dislocation. On the other hand, we observe here that the oxygen vacancies can reside both in the tensile and in the compressive zones, as well as in the dislocation core, simply following the trivalent dopant distribution. This is because of electrostatic attraction of the positively charged oxygen vacancies to the negatively charged dopant cations. From the picture described above, it appears that the dislocation strain field attracts the differently sized trivalent dopants based on elastic interactions, and the trivalent dopants attract the oxygen vacancies based on electrostatic interactions, leading to a segregation profile of both types of defects at the same location. To confirm this, we decouple the dopant–vacancy interaction from the dislocation–vacancy interaction, by studying a hypothetical model, hereafter referred to as h-CeO 2− δ . In h-CeO 2− δ , when vacancies are introduced (that is, δ >0), charge compensation is achieved by simply assigning all the cerium cations with the same valence and size (see Supplementary Methods for the details). This approach has been used in previous work to decouple the dopant–vacancy interaction from other point defect interactions [50] . Although this model is not a physically realistic one (thus the name ‘hypothetical’), it allows us to isolate certain interactions among defects in a way that is not possible to do experimentally. In this model, as all the cations are equal in size, no elastic interactions remain between any of the cations and the dislocation. In the absence of cation segregation in the h-CeO 2− δ model, vacancy segregation still takes place ( Fig. 3a ). At 700–1,300 °C, oxygen vacancies enrich in the three oxygen columns, which directly face the dislocation core, and they deplete in three petal-shaped zones next to the enrichment zones. This picture displays the outcome of the vacancy–dislocation interaction alone. Next, by comparing Fig. 2e–h with Fig. 3a , we can see that the redistribution profile of vacancies is more narrowly confined and not exceeding a spread over of 1 nm radius, with oxygen vacancies concentrated at the oxygen lattice sites at the dislocation core. The highest intensity of oxygen vacancies at the core sites (6%) is comparable to that in the broader enrichment zones of the realistically doped ceria models described above. The enrichment sites are surrounded by three separate depletion zones of ~1 nm wide. This drastic difference in the vacancy profiles confirms that the enrichment and depletion of oxygen vacancies near the dislocation in the realistically doped ceria is driven mainly by the dopant–vacancy interactions and not by the vacancy–dislocation interaction alone. 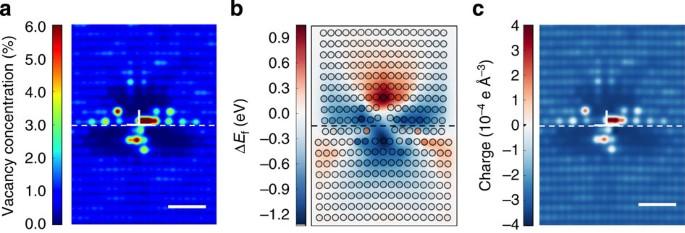Figure 3: Distribution of oxygen vacancies and net charge in h-CeO2−δ. For the hypothetical ceria model, h-CeO2−δ(δ=0.04), the nominal vacancy concentration is 2%, which is equivalent to those in 8% doped CDC, GDC, YDC and SDC. (a) The equilibrated distribution of oxygen vacancies at 900 °C. Dashed line marks the location of the glide plane. (b) The spatial map of the formation energy of a single oxygen vacancy at each site around the dislocation core, with the dislocation at the centre of the plot. (c) The net charge profile for h-CeO2-0.04at 900 °C, which follows the same pattern as ina. Scale bar, 1 nm. Figure 3: Distribution of oxygen vacancies and net charge in h-CeO 2− δ . For the hypothetical ceria model, h-CeO 2− δ ( δ =0.04), the nominal vacancy concentration is 2%, which is equivalent to those in 8% doped CDC, GDC, YDC and SDC. ( a ) The equilibrated distribution of oxygen vacancies at 900 °C. Dashed line marks the location of the glide plane. ( b ) The spatial map of the formation energy of a single oxygen vacancy at each site around the dislocation core, with the dislocation at the centre of the plot. ( c ) The net charge profile for h-CeO 2-0.04 at 900 °C, which follows the same pattern as in a . Scale bar, 1 nm. Full size image For the same hypothetical model, h-CeO 2− δ , a spatial map of oxygen vacancy formation energy is plotted in Fig. 3b . The formation energy is lowest at the tensile zone close to the dislocation core (marked as bluest dot in Fig. 3b ) and it is highest at the compressive strain zone. In metals, the structural relaxation around a vacancy can release the strain in the compressive zone and hence lead to smaller formation energy [51] . However, in ceria, an ionic material with strong bonds, the bond breaking during the vacancy formation plays a key role in determining the vacancy formation energy. The bonds in tensile zone are longer, weaker and easier to break than the compressive zone, so that the formation energy is lower in the tensile zone around the dislocation. This trend is consistent with the effect of uniaxial strain along [110] in bulk (dislocation free) ceria, where the formation energy of oxygen vacancy is higher by 0.38 eV with −2.5% (compressive) and lower by 0.43 eV with 2.5% (tensile) strain (see Supplementary Fig. 2 ). The positions of lowest formation energy in Fig. 3b match well with the zones where vacancies accumulate, as shown in Fig. 3a . The depletion in Fig. 3a is, however, stronger than that predicted by oxygen vacancy formation energy shown in Fig. 3b . The reason is that at 2% vacancy concentration, in addition to the vacancy–dislocation interaction, the electrostatic interactions among vacancies and the interaction of the vacancies with the negatively charged background (2 δ - per cation) also need to be considered. As this model has a uniform and equal charge distribution on each cerium cation (2 δ - per cation) with positively charged oxygen vacancies (2+ per vacancy), the enrichment of oxygen vacancies induces a positively charged dislocation core, accompanied by the formation of depletion zones that are negatively charged around the dislocation (the petal-shaped dark zones surrounding the bright columns at/near the dislocation core). This charge separation presents a direct atomistic simulation and visualization of the space charge region of the dislocation in h-CeO 2− δ ( Fig. 3c ). Net charge of the dislocation in doped or reduced ceria The segregation profiles of trivalent cations and positively charged oxygen vacancies, shown in Fig. 2a–h , raise the question of whether there exists extensive space charge zones around the dislocation in the realistically doped or reduced ceria models. Space charge is often invoked when interpreting experimental results on oxygen diffusion kinetics [52] , [53] ; hence, this question is of interest. The dislocation core and strain fields can be charged either positively by an exceeding amount of oxygen vacancies or holes, or negatively by an exceeding amount of aliovalent dopants or electrons. In Fig. 2i–l we present our calculated net charge distribution. The positively charged regions and its adjacent negatively charged regions are as small as one lattice site on the dislocation core. These ‘charged’ regions are simply a consequence of the discreet nature of crystals, with alternating positively and negatively charged atomic planes, and could not be called a space charge region. In addition, in contrast to the observed 1–2 nm extent of the dopant or vacancy segregation in the real ceria models (see Fig. 2a–h ), the extent of charge separation is very small. A larger charged region is present only in the h-CeO 2− δ system ( Fig. 3c ), which is exactly the same as the segregation profile ( Fig. 3a ). We recall here previous experimental studies that found evidence to the enrichment of dopant cations and oxygen vacancies at or near the grain boundary of ceria [54] , [55] . Those findings appear consistent with the segregation profiles we predict near the edge dislocation. However, despite the enrichment profiles found in those previous experiments, it is not clear whether a space charge layer is formed near the grain boundary. Space charge layer is a consequence of the electrostatic interaction between the extended defects and the point defects. The associative interactions between the point defects themselves are usually neglected in these space charge models, because they assume a dilute concentration of defects. However, the charged defect redistribution around the edge type 1/2 {100}<110> dislocation in our model is caused primarily by the elastic energy minimization in the strain field. When the system is reaching equilibrium, the differently sized cations (or negative charge) accumulate in their respective strain fields and the positively charged oxygen vacancies follow the dopants that ultimately neutralize the strain fields of the dislocation. At such high concentrations of point defect (dopant concentration>8%), the interaction between the dopants and oxygen vacancies is non-negligible. It is also known that the space charge zone width is proportional to the , where [ c ] is the defect concentration [34] , [56] . For these reasons, it is reasonable that the redistribution of point defects in the realistic doped ceria model at large concentration of defects around the dislocation does not result in extensive space charge regions. The redistribution of Ce 3+ and oxygen vacancies in reduced ceria is also examined by DFT+U calculations here. Ce 3+ in reduced ceria is actually a polaron with a low hopping barrier of 0.4 eV [57] . Accumulation of polarons in the dislocation may, in principle, form delocalized electronic states at the dislocation core. This scenario is impossible to be modelled by classical potentials whose results were presented above. From the DFT calculations, we find that the oxygen vacancy formation energy is lower in the tensile zone and higher in the compressive zone (summarized in Supplementary Table 1 ), qualitatively consistent with Fig. 3b derived from classical potentials. Furthermore, oxygen vacancy formation at the core of 1/2<110>{100} edge dislocation in ceria was found to be always compensated by two polarons well localized on two cerium cations. This is shown in Fig. 4 ; the two polarons are localized separately at two cerium cations when one oxygen vacancy formed at the dislocation core. There is no evidence to electron delocalization into/along the dislocation core that would make it a negatively charged dislocation core. 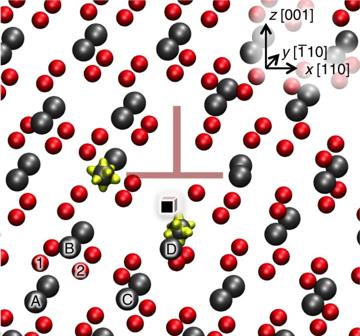Figure 4: Position of polarons on oxygen vacancy formation in ceria with a dislocation. The spin density of reduced ceria with an oxygen vacancy formed at the core of the edge dislocation, calculated by DFT+U. The black cube marks the position of oxygen vacancy. The spin density difference is shown as the yellow clouds localized on to cerium cations near the vacancy. The two polarons (letters) and oxygen vacancies (numbers) arranged as A-B-1, A-D-1, A-D-2 and B-C-2 are also calculated, as summarized inTable 1. Figure 4: Position of polarons on oxygen vacancy formation in ceria with a dislocation. The spin density of reduced ceria with an oxygen vacancy formed at the core of the edge dislocation, calculated by DFT+U. The black cube marks the position of oxygen vacancy. The spin density difference is shown as the yellow clouds localized on to cerium cations near the vacancy. The two polarons (letters) and oxygen vacancies (numbers) arranged as A-B-1, A-D-1, A-D-2 and B-C-2 are also calculated, as summarized in Table 1 . Full size image To assess where the Ce 3+ cations prefer to reside in the strain field of the dislocation, we also calculated the relative formation energy of different arrangements of polarons and oxygen vacancies (see Table 1 and Fig. 4 ). The configurations are shown as A-B-1, A-D-1, A-D-2 and B-C-2 in Fig. 4 , where the letters denote the position of the polaron and the numbers denote the position of the oxygen vacancy. The results show that the polarons prefer to stay at site D—the position closest to the core in the tensile strain field of the dislocation, rather than residing at the nearest neighbour site of the oxygen vacancies (A, B or C). This indicates that in reduced ceria, elastic energy minimization drives Ce 3+ segregation around the dislocation. These results deduced from DFT calculations validate our results from the classical potential simulations for locating the position of Ce 3+ cations near the dislocation in the CDC model. Table 1 Relative oxygen vacancy formation energy* at different sites around the edge dislocation. Full size table Slow oxygen diffusion along the dislocation The impact of the 1/2<110>{100} edge dislocation on oxide ion conductivity is studied by molecular dynamics simulations. This is presented here for three scenarios: (1) the 8% doped or reduced ceria (equivalently 2% oxygen vacancy concentration) upon obtaining the equilibrated distribution of dopants and oxygen vacancies by MCMD calculations (as in Fig. 2 ); (2) the hypothetical model system, h-CeO 2− δ , upon obtaining the oxygen vacancy redistribution profiles (as in Fig. 3 ); and (3) a non-equilibrium scenario with random distribution of dopant cations. This last model represents a meta-stable state, for example, oxide thin films fabricated at low temperature, which does not allow enough time for the cations (which have high migration energies in the bulk [58] ) to equilibrate. In all three models we find that, compared with bulk, there is no enhancement of oxygen diffusivity induced by the dislocation. This finding is also valid for every composition and concentration level studied in this study, including 4%–12% CDC and 4%–12% GDC ( Supplementary Fig. 3 ). To uncover whether the dislocation serves as a fast ‘pipe’ pathway, one-dimensional oxygen diffusivity along the dislocation line is analysed, instead of three-dimensional diffusivity as those in bulk. We also show in Supplementary Movie 1 that the diffusion properties of the dislocations can be anisotropic: during the molecular dynamics simulation of a 8% GDC system at 900 °C (3–5 ns), the oxygen vacancies rarely hop out of the dopant enrichment zone or diffuse across the dopant depletion zone, while in the region far away from the dislocation, the vacancies diffusion is isotropic. This video demonstrates the trapping nature of dislocations, which would slow down the oxygen diffusion across the dislocation. The one-dimensional diffusivity is defined as where ‹ s i 2 › is the mean square displacement of oxide ions along the direction i and t is the time needed for this displacement. The diffusion along the x , y and z directions (see Fig. 1 ) represent the diffusion across the dislocation parallel with the glide plane, along the dislocation and across the dislocation normal to the glide plane, respectively. 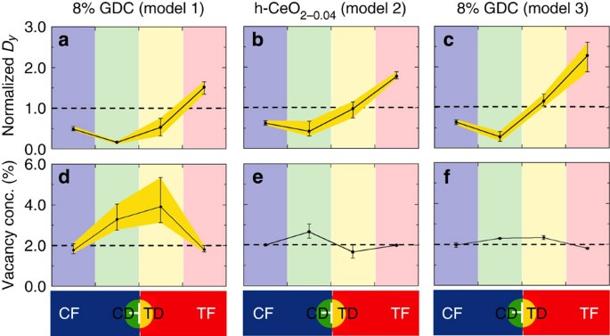Figure 5: Local oxide ion diffusivity and vacancy concentration. Local oxide ion diffusivity along the dislocation, and local oxygen vacancy concentration near and far from the dislocation at 900 °C: (a,d) Model 1 of 8% GDC with equilibrated dopant cation distribution. (b,e) Model 2 of 2% vacancy concentration in h-CeO2-0.04(equivalent to the oxygen vacancy concentration in Model 1). (c,f) Model 3 of 8% GDC with random distribution of dopant cations. The geometry of the four regions for each of the three models is shown in the schematic plot below each column and colour coded in the online version (yellow for the TD region and green for the CD region, red for the uniaxial tensile region far from dislocation (TF), blue for uniaxial compressive region far from dislocation (CF)). Three to five samples were calculated for each model. The error bar indicates the maximum and minimum diffusivity or oxygen vacancy concentration found in these samples. Figure 5 shows the computed diffusivity along the dislocation, D y , normalized by the one-dimensional diffusivity in the bulk ceria model with the same nominal composition. Figure 5: Local oxide ion diffusivity and vacancy concentration. Local oxide ion diffusivity along the dislocation, and local oxygen vacancy concentration near and far from the dislocation at 900 °C: ( a , d ) Model 1 of 8% GDC with equilibrated dopant cation distribution. ( b , e ) Model 2 of 2% vacancy concentration in h-CeO 2-0.04 (equivalent to the oxygen vacancy concentration in Model 1). ( c , f ) Model 3 of 8% GDC with random distribution of dopant cations. The geometry of the four regions for each of the three models is shown in the schematic plot below each column and colour coded in the online version (yellow for the TD region and green for the CD region, red for the uniaxial tensile region far from dislocation (TF), blue for uniaxial compressive region far from dislocation (CF)). Three to five samples were calculated for each model. The error bar indicates the maximum and minimum diffusivity or oxygen vacancy concentration found in these samples. Full size image The normalized one-dimensional local oxygen diffusivities ( D y ) along the dislocation ( y axis) at 900 °C in different regions of the three models are plotted for: (1) GDC with dopant cations equilibrated at 1,300 °C before the molecular dynamics calculations ( Fig. 5a ); (2) h-CeO 2− δ model with 2% of oxygen vacancies (equivalent to the vacancy concentration in models 1 and 3) also equilibrated at 1,300 °C before the dynamic simulations ( Fig. 5b ); and (3) 8% GDC with random distribution of Gd 3+ ( Fig. 5c ). Four different regions were analysed in the models, including two regions that are at tensile or compressive strain fields of the dislocation with a semi-cylindrical volume of diameter 3 nm and two regions far away from the dislocation with uniaxial tensile or uniaxial compressive strain. These regions are labelled as TD, CD, TF and CF, respectively, in the schematics in Figs 1 and 5 . The limited size of TD and CD in the direction of x and z leads to relatively poor statistics of D x and D z , which are not plotted here. Instead, the effect of dislocation can be qualitatively shown in the Supplementary Movies 1 and 2 , where it is possible to observe that the diffusion of oxide ions along x and z directions is hindered by the dislocation. One can see clearly in Fig. 5a–c that D y in all of the dislocation zones (average of D y in TD and CD) is smaller than the unstrained bulk D y (shown as a dashed reference line) in these simulated models that comprehensively span a wide range of compositions and scenarios. In the GDC and h-CeO 2− δ models, both the TD and the CD zones have slower oxygen diffusivity compared with bulk. In the zones far from the dislocation in all three models, the local diffusivity depends on the local uniaxial strain. The highest local diffusivity is observed at the tensile zone (TF), around 1.5 times compared with the unstrained bulk. At the same time, the diffusivity is much lower in the compressive strain zone (CF). The concentrations of oxygen vacancies in these zones away from the dislocation are close to 2% ( Fig. 5d–f ), not affected by the dislocation. The higher diffusivity in the TF zone and lower diffusivity in CF zone is in agreement with previous computational studies that found elastic tensile strain to accelerate oxide ion conductivity in related materials [11] , [59] , [60] . For model 1 with equilibrated distribution of Gd 3+ ( Fig. 5a ), the normalized D y at the TD zone and CD zone are 0.5 and 0.3 on average, respectively, significantly lower than that in the unstrained bulk. A similarly low local diffusivity is also observed in the proximity of the dislocation even for model 2, the h-CeO 2− δ ( Fig. 5b ). In this model, although there is no segregation of different cations, vacancy enrichment and depletion zones were shown in Fig. 3 . Here, the CD and CF zones all have diffusivities lower than a half of the unstrained bulk. TD has a diffusivity comparable to bulk diffusivity (normalized D y ~1), despite the large concentration of vacancies, suggesting that mobility of oxygen vacancies is again low. For model 3 ( Fig. 5c ), the oxygen vacancies and with Gd 3+ dopant cations are uniformly distributed over the volume, as indicated in Fig. 5e , with a 2% vacancy concentration across all four zones. Although the tensile strain in the TD zone of the dislocation slightly enhances the oxide ion diffusivity to 1.2 times that of the unstrained bulk, the compressive strain in the CD zone depresses the oxygen diffusion with diffusivity as low as 0.3 times of the bulk diffusivity. Therefore, there is effectively no gain from the presence of a dislocation also in this model. As noted above, the slow diffusion of oxide ions presented in Fig. 5 was also found, with varying magnitudes, in 4%–12% CDC, 4%–12% GDC and 8% YDC ( Supplementary Fig. 3 ). This result confirms that edge dislocations do not enhance the ionic conductivity of these materials, regardless of the cation type or distribution. This is counter to what is known in metals, where dislocations serve as fast pipe pathways for atoms. The impact of edge dislocations in slowing down the oxide ion conduction found in ceria can be explained by the segregation of charged defects, driven by the elastic strain field of the dislocation along with the electrostatic and elastic interactions among the charge defects. For the equilibrated samples of model 1, exemplified by GDC with segregation of dopants and oxygen vacancies, and of model 2, the h-CeO 2− δ with segregation of oxygen vacancies alone, the slow oxide ion transport along the dislocation originates from the associative interactions among the charged point defects. It is well known that in doped ceria, the bulk diffusivity has a nonlinear dependence on the dopant concentration: the diffusivity increases up to a maximum value with increasing concentration of dopants till 8%–10% and decreases at higher dopant concentrations [61] . At low doping concentration, the lack of oxygen vacancies and thus a low concentration of charge carriers reduce the diffusivity. At high doping concentration, strong vacancy–vacancy repulsion and vacancy–dopant association effects increase the migration barriers for oxygen vacancies, and thus are the reason for low diffusivity [36] , [50] , [62] , [63] . In the models simulated in this study, although the average dopant concentration is at the optimum value of 8% over the whole slab, the local concentration around the dislocation significantly deviates from this value, as was shown in Fig. 2a–d . The found significant segregation then takes the system locally away from the optimal composition. In model 1, in the TD zone and at the columns directly facing the dislocation core in the CD zone, the high density of dopant cations and oxygen vacancies blocks the oxide ion diffusion. On the other hand, the compressive strain in the CD zone depletes the oxygen vacancy concentration and the subsequent lack of vacancies decreases the local oxygen diffusion. Therefore, both the TD and CD zones slow down the oxygen diffusion. In model 2, the h-CeO 2− δ , oxygen vacancies move around the dislocation without any dopant–vacancy interaction. However, the oxide ion transport still suffers from the strong vacancy–vacancy interaction in the enrichment zone and the lack of charge carriers in the depletion zone, similar to the realistically doped case in model 1. When dopant cations are randomly distributed in the doped ceria, for example, 8% GDC as model 3 in Fig. 5c , the only factor that remains to influence the oxygen diffusion is the strain field of the dislocation. The large tensile strain around the dislocation was found to slightly facilitate the oxygen diffusion. The compressive strain around the dislocation depresses the diffusion. It seems that the large magnitude of tensile (but distorted) strain field around the dislocation (as shown in Fig. 1 ) does not help diffusion as much as the (smaller) uniaxial tensile strain condition far from the dislocation. Overall, the strain–stress field of the dislocation leads to no enhancement of the overall oxygen diffusion along the dislocation (averaging the TD and CD zones). The mechanism responsible for the slow diffusion along an edge dislocation in ceria is quite different from those observed in uranium dioxide [43] , alumina [64] and magnesium oxide [65] , in which dislocations were found to be fast pipe diffusion paths. For uranium and alumina, the fast ion diffusion at dislocations is mediated by interstitial type oxygen defects. The open space at the dislocation core can offer a fast diffusion channel to these interstitials by reducing their migration energy as well as increasing their concentration. For alumina and magnesium oxide, the low concentration of defects in their bulk (p.p.m. levels of oxygen vacancies and interstitials, which is lower by many orders of magnitude than the defect concentrations found in ceria [36] ) results in small bulk diffusion coefficients. Therefore, the interactions among these point defects are negligible. A slight reduction in the formation energy of oxygen defects due to strain field or open space can lead to a higher concentration at/near the dislocations in alumina or magnesium oxide compared with bulk, and subsequently a faster diffusion along the dislocation at low temperatures. Our results can be generalized to oxides, which have dopant concentration levels that are of the same order of magnitude as those in this paper. We cannot extrapolate our current results to oxides that are only dilutely doped, for example, at p.p.m. level in bulk. In summary, the influence of edge dislocations on the oxide ion conductivity in reduced and doped ceria was studied by atomistic simulations. In general, a slower oxide ion transport is present along the edge dislocation in these materials. The strain field drives dopants to segregate around the dislocation, building enrichment and depletion zones. This dopant redistribution subsequently drives the segregation of oxygen vacancies with the same profile, due to the electrostatic interactions. The local dopant concentration in the enrichment zone near the dislocation can be as high as 30%, which is much greater than the optimum doping concentration for maximum conductivity in doped ceria. Therefore, the strong dopant–vacancy and vacancy–vacancy interactions slow down oxide ion diffusion in the enrichment zone. On the other hand, the lack of oxygen vacancies in the defect depletion zone around the dislocation also reduces the oxide ion conductivity. If the system is meta-stable, that is, the dopants and oxygen vacancies are uniformly distributed without a segregation profile around the dislocation, then the compressive strain field reduces the mobility, while the tensile field of the dislocation increases the mobility to a small extent. Overall, even in such a meta-stable case, the dislocation does not enhance the oxide ion conductivity. We believe these results and mechanisms are generally applicable to other doped or reduced oxide ion conductors with defect concentrations on the same order of magnitude as studied for ceria here. For example, in YSZ, oxygen transport is also mediated by oxygen vacancies, Y 3+ cation has a large size compared with the Zr 4+ cation and the diffusivity depends on the Y 3+ concentration nonlinearly, with a peak around 16% of Y 3+ (ref. 66 ). Therefore, segregation and diffusion profiles obtained for model 1 in this paper are expected to be valid also for YSZ. The hypothetical model (model 2) can be conducive to the oxide materials where the charge of oxygen vacancies is compensated by delocalized electrons, for instance, as in strontium titanate [17] . Overall, the decisive factor is the dislocation’s strain field and the defect chemistry of the material. A strong strain field around the dislocation can attract or repel the charged defects and, consequently, the excessive accumulation or depletion of charge carriers, both, decreases the local diffusivity. This understanding of dislocations is important in quantitatively interpreting the experimental results aiming to assess the effects of strain in oxygen conductivity in ionic solids. Furthermore, due to the ubiquitous nature of dislocations in thin films and their importance in several technological applications, such as SOFCs, resistive switching and ferroelectrics, this fundamental understanding can be used by researchers to engineer the properties of materials for these devices. Atomistic simulations with classical potentials Classical molecular dynamics simulations were performed by using the LAMMPS package [67] . The employed inter-ionic potential was a rigid ion model combining a coulombic interaction with a short range Buckingham term, with a cut-off radius of 10 Å [68] . This potential is able to describe the lattice parameter for reduced ceria, GDC, YDC and SDC, and the nonlinear dependence of the oxygen diffusivity on the dopant concentration in the bulk CDC and GDC. Details are available in Supplementary Figs 4 and 5 , Supplementary Table 2 and 3 , and Supplementary Methods . Setting up a slab of ceria with an ½<110>{100} edge dislocation The ½<110>{100} edge dislocation was introduced to the slab with {100} surfaces by the following steps: (1) create a slab of ceria with x , y and z axes along [110], and [001] directions, respectively. (2) Remove a lattice plane from the bottom half of the slab, from x =½ L x to and from z =0 to z =½ L z , where a is the lattice parameter, Lx and Lz are the width and thickness of the slab along the x and z axes. This is shown in Supplementary Fig. 6a . (3) Perform a conjugate-gradient (CG) structural optimization. As seen in Supplementary Fig. 6b , the empty slit in the bottom half of the plane was ‘healed’ by this CG structural optimization. An edge dislocation along [110] direction, lying on the {100} plane was thus formed at the centre of the slab, however, with an asymmetric meta-stable core structure. This is because of the asymmetric geometry of the as-constructed structure, shown in Supplementary Fig. 6a . (4) Anneal the supercell for 100 ps at 1,000 °C by MD simulation and perform another CG optimization. This last step allows for achieving the ground state of the core structure. As seen in the Fig. 1a in the paper, the oxygen anion column along [110] direction in the dislocation core is split into two columns. This symmetric dislocation core structure has the lowest potential energy, lower than the asymmetric one shown in Supplementary Fig. 6b . Electrostatic potential energy of each oxygen ion around the ground-state dislocation can also be seen in Supplementary Fig. 7 . This system was periodic along the x and y directions but non-periodic along the z direction, and consists of about 26,000 atoms. The surfaces of the slab were constructed as non-polar surfaces with {100} half-filled oxygen terminations. Because of the way we constructed the dislocation and with periodic boundary conditions along [110] and directions, the top part of the slab has one lattice plane more than the bottom part. As a result, the top and bottom of the slab are strained uniaxially along [110] at 2.5% compressive strain and 2.6% tensile, respectively. Both surfaces reconstruct after relaxation. The surface reconstruction after CG optimization and 100 ps MD at 1,000 °C are shown in Supplementary Fig. 6c–h . The compressive strain at the top surface led to a strong reconstruction on the top two oxygen planes and cerium planes were reconstructed, whereas for the surface with tensile strain the top layers contracted towards the bulk to further reduce the surface polarization. These two surfaces in our system show segregation of both cations and oxygen vacancies, in agreement with previous studies [40] . The spatial extension of this segregation layer is, however, limited to 1–2 nm from the top and bottom surfaces, so that the surface does not have any impact in the vicinity of dislocation; the dopant segregation profile near the surfaces can be found in Supplementary Fig. 8 . Hybrid MCMD algorithm An MCMD algorithm [39] , [40] was coded into LAMMPS in this work. This algorithm was used to equilibrate the dopant distribution by MC simulation and the oxygen vacancy distribution by MD simulation. In each MC trial move, a dopant cation was randomly selected and was swapped with another randomly selected host cation. The trial move is accepted with a probability within min{1, exp(−Δ E / k B T )}, where Δ E is the change of system energy and T is the temperature (in this work, T =1,300 °C). Δ E in this work is calculated after a CG structure optimization that allows the neighbouring ions to relax, once the cations have been swapped; a slightly different step than that implemented in references [39] , [40] . Starting with a random and uniform distribution of trivalent cations and oxygen vacancies, an equilibrium cation and vacancy distribution was obtained by performing ~10 5 attempted MC trial moves, with 6,000 of them accepted, and 6 ns of MD simulation (we performed a 100 ps of isothermal-isobaric (NPT) MD run after every 100 successful MC moves). The results of defect distributions shown in Fig. 2 were obtained by averaging over the last 3,000 successful trial moves from 3 initial configurations for each composition and concentration level. Mean square displacement calculation The oxide ion diffusion coefficients were calculated from the slope of their mean square displacements, obtained from long (>3 ns) MD simulations. For each composition and concentration level, the diffusion coefficient is found by averaging over three to five independent MD calculations (details in Supplementary Fig. 9 and Supplementary Methods ). DFT calculations The DFT calculations reported in this study were performed with the VASP code [69] , within the projector augmented wave method. We used the generalized gradient approximation with the Perdew-Wang 91 exchange-correlation functional and an energy cutoff of 400 eV. A Hubbard (+U) correction, with U =5 eV, was added to properly model the localized character of the 4 f electrons [70] . All the calculations were carried out using the Brillouin zone sampled with a (1 × 2 × 1) Monkhorst–Pack mesh k -points grid. Further details can be found in the Supplementary Fig. 10 and Supplementary Methods . How to cite this article: Sun, L. et al. Edge dislocation slows down oxide ion diffusion in doped CeO 2 by segregation of charged defects. Nat. Commun. 6:6294 doi: 10.1038/ncomms7294 (2015).